Carbene-catalyzed chemoselective reaction of unsymmetric enedials for access to Furo[2,3-b]pyrroles A carbene-catalyzed chemoselective reaction of unsymmetric enedials is disclosed. The reaction provides a concise access to bicyclic furo[2,3-b]pyrroles derivatives in excellent selectivity. A main challenge in this reaction is chemoselective reaction of the two aldehyde moieties in the enedial substrates. Mechanistic studies via experiments suggest that our chemoselectivity controls are mostly achieved on the reducing properties of different sited Breslow intermediates. Several side reactions processes and the corresponding side adducts are also studied by high resolution mass spectroscopy analysis. Our method allows for efficient assembly of the furo[2,3-b]pyrrole structural moieties and their analogues widely found in natural products and pharmaceuticals. Chemoselective reactions of two or multiple functional groups with similar reactivities remain an ongoing challenge in chemistry. Some of such selectivity issues may be addressed (in industrial practices) through the use (and recycle) of certain reagents in large excess. On the other hand, it is much more attractive both scientifically and practically to achieve selective reactions in the first places. Organic catalysis has been proven to be a versatile approach for activation and selective controls [1] , [2] , [3] , [4] , [5] . Much attention have been placed to modulate the steric interactions between the catalysts and substrates to achieve selective controls (Fig. 1a ) [6] , [7] , [8] , [9] . N-heterocyclic carbene (NHC) catalysts [10] , [11] , [12] , [13] , [14] provide unique activation and reaction modes for a diverse set of reactions, and impressive reactions with selectivity modulated mostly by steric interactions have been widely studied [15] , [16] , [17] , [18] , [19] . Furthermore, it is well explored that the Breslow intermediates can be oxidated by various oxidants [20] , [21] , [22] , [23] , [24] , [25] , [26] , [27] , [28] , [29] , [30] , [31] . However, the high chemoselectivity is mainly controlled via redox (rather than steric) properties of the substrate/catalyst remains undeveloped to date. It appears to us the redox properties brought by both the NHC catalysts and the reacting substrates can be explored to achieve unusual reaction controls (Fig. 1a ). Specifically, in such a scenario, turning the redox properties of catalysts and substrates/reagents can likely have profound effects on the reaction outcomes [32] , [33] , [34] , [35] . Fig. 1: Selective reactions of unsymmetric enedial. a Approaches for selective controls. b Selective oxidation via redox event. Full size image In this work, we develop a chemo- and enantioselective strategy transforming unsymmetric enedials to furo[2,3-b]pyrrole containing molecules. The overall chemoselectivity observed is due to an oxidation event of the Breslow intermediate which provides a very significant increase to the chemoselectivity. Chemoselective reactions of unsymmetric enedials can be achieved through an oxidative process (Fig. 1b ). Mechanistic studies via high-resolution mass spectroscopy (HRMS) suggest that our process is chemoselective during two of the key steps. With imine [36] , [37] , [38] , [39] as the other reaction partner, our chemoselective reactions of unsymmetric enedials afford bicyclic furo[2,3-b]pyrroles derivatives in excellent diastereo- and enantioselectivity with the formation of four new chemical bonds and two chiral centers. Our findings can likely stimulate further explorations for unique reactions by placing more attentions on the redox steps of many organic catalytic reactions. Reaction development Our study provides a much less explored strategy via a redox process in achieving otherwise challenging chemoselectivity. Further development via similar logics is expected to bring surprises in reactions controls. In the model reaction, the addition of NHC catalyst to the enedial leads to the formation of Breslow intermediate between the NHC catalyst and the enendial substrate did not provide sufficient differentiations (Fig. 1b ). Subsequently, it was the chemoselectivity determining step that the oxidation of the Breslow intermediates to form the α, β-unsaturated acyl azolium intermediates 1a(D) - II and 1a(D) - II’ . In the redox step, the two intermediates 1a(D) - II and 1a(D) - II’ exhibit excellent chemoselectivity ratio 99:1. Then the acyl azolium intermediate 1a(D) - II reacted with imine to form the final chiral furo[2,3-b]pyrrole containing products with high optical purities. Such furo[2,3-b]pyrrole is a common structural motif widely found in natural products and pharmaceuticals, such as diazonamide, physovenine and quinamine (Fig. 2 ) [40] , [41] , [42] , [43] , [44] , [45] , [46] , [47] , [48] , [49] , [50] . 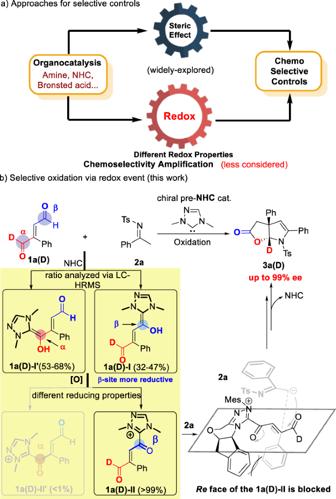Fig. 1: Selective reactions of unsymmetric enedial. aApproaches for selective controls.bSelective oxidation via redox event. Key results of the optimization of the reaction conditions are summarized in Table 1 . Enedial 1a was selected to react with imine 2a under the catalysis of various pre-NHC catalysts (Table 1 , entry 1 to 3, respectively). We found that pre-catalyst A bearing a 2,4,6-trimethylphenyl (Mes) group, gave the product 3a in a moderate yield and 96:4 er (Table 1 , entry 1). The enantioselectivity could be enhanced by switching bases, and 3a was obtained in 51% yield and 97:3 er by using K 2 CO 3 (Table 1 , entry 5). In addition, the solvents had a strong impact on reactions, switching THF to MeCN gave the 66% yield and the excellent enantioselectivity (98:2 er) with 4 Å molecular sieves (MS) as an additive (Table 1 , entry 12). Furthermore, we evaluated different sterically hindered oxidants, it was found no obviously erosion of the er values and the yields when the bulky less oxidants were employed (Table 1 , entry 13, 14). The product 3a formed in this chiral catalytic process was isolated as a single diastereomer. Fig. 2: Functional molecules containing furo[2,3-b]pyrrole. Examples of functional chiral molecules. Full size image Table 1 Initial studies and reaction optimization a Full size table Substrate scope Having established acceptable reaction conditions, we evaluated the generality of the reaction using substrates enedial 1 and imine 2 with different substitutions (Fig. 3 ). Initially, we studied the reaction scope of enedials 1 . Both electron-withdrawing and electron-donating substituents could be installed on each (para-, meta- or ortho-) position of benzene ring of the enedials substrate 1 , with the corresponding products afforded in moderate to good yields with high optical purities (Fig. 3 , 3a – 3i ). Alkyl enedials substrates were not be synthesized by general procedure, which was mentioned in supporting information. We will further investigate this problem in our further studies of this class of molecules in relevant application-driven projects. The catalytic approach could also be carried out at 1.0 mmol scale with the desired product 3a afforded in good yield and excellent enantioselectivity (258.9 mg, 60%, 97:3 er). We then moved to examine the reaction scope of imine as substrates 2 with enedial 1a (Fig. 3 ). It was found that both electron-withdrawing and electron-donating substituents were well tolerated ( 4a – 4o ), and the desired products were produced in moderate to good yields and excellent enantioselectivities. The benzene ring of the imine could also be replaced with naphthalene group and the desired product 4p was produced in good yield and high enantioselectivity. The substituted benzene moiety of the imine could be exchanged to heteroaromatic moieties without erosion of enantioselectivities and the yields of corresponding products were enhanced ( 4q – 4r ). It is worth noting that aliphatic imines could also be used as suitable reaction substrates in this reaction, with the desired product 4 s and 4t afforded in moderate yields and excellent enantioselectivities. The er value of the product 4t decreased slightly when a tert-butyl imine was used as the substrate, this may be caused by the steric hindrance. Fig. 3: Substrates scope of the reaction a . a Reaction conditions as stated in Table 1 , entry 12. Yields were isolated yields after purification by column chromatography. Er values were determined via HPLC on chiral stationary phase. b The reaction was carried out at 1.0 mmol scale based on 2a . Full size image Synthetic transformations Additionally, the chiral furo[2,3-b]pyrrole containing product 3a was easily transformed into various derivatives through simple protocols (Fig. 4 ). For instance, the hydrogen atom of 3a was employed to react with N-bromo-succinimide (NBS) (2 eq), the brominated product 5 was obtained in 87% yield and 99:1 er. Increasing the loading of NBS (up to 10 eq), the dibromo product 8 could be isolated with high optical purity. Moreover, switching NBS to N-chloro-succinimide (NCS), the dichloride product 6 could be obtained in good yield and excellent er value. In addition, compound 7 could be synthesized when using triphenylphosphine to reduce the dichloride product 6 . The absolute configuration of products was determined by X-ray diffraction analysis. The 3a could be completely reduced with Mg/MeOH to give the diphenyl substituted pyrrole 9 in 76% yield. Fig. 4: Synthetic transformations of 3a. Derivatization studies on 3a . Full size image Mechanistic studies To understand the mechanism of the reaction, some mechanistic studies were performed. The deuterium labeled (abbreviated as D-labeled) α - aldehyde moiety substrate 1a(D) was synthesized, then 1a(D) was reacted with imine 2a in the model reaction condition (Table 1 , entry 12). Finally, the D-labeled product 3a(D) was obtained in 66% yield and 98:2 er (Fig. 5a ), the reaction results were similar to non-deuterium labeled model reaction. It suggested that the D-labeled 1a(D) can be used as model substate to study the driving force of chemoselectivity in reactions. Fig. 5: Additional supporting mechanistic experiments. a Model reaction of 1a(D) . b Intensity of Breslow intermediates via LC-HRMS. c Intensity of acyl azolium intermediates via LC-HRMS. d DFT calculation for the oxidation process. e Possible polymerized product analyzed by HRMS. Full size image The carbene catalyst addition to one of the two aldehyde moieties of 1a(D) to form two type Breslow intermediates 1a(D)-I and 1a(D)-I’ (Fig. 5b ), the D-labeled Breslow intermediate 1a(D)-I was one Dalton greater than the non-labeled Breslow intermediate 1a(D)-I’ , the differentiation of the molecular weight can be determined via in situ liquid chromatography high resolution mass spectroscopy (LC-HRMS), it means that the reacted site can be clearly confirmed. Furthermore, the response intensity of the D-labeled and non-labeled Breslow intermediates was detected and differentiated by LC-HRMS. It was found that the intensity ratio of 1a(D)-I and 1a(D)-I’ was (32-47%):(53-68%), which means that the β-aldehyde moiety was more favorably reacted with NHC catalyst. Subsequently, the selective redox of Breslow 1a(D)-I and 1a(D)-I’ was studied. Base on the model reaction, 3,3’,5,5’-tetra-tert-butyl-[1,1’-bi(cyclohexylidene)]−2,2’,5,5’-tetraene-4,4’-dione (DQ A) was added to oxidize the Breslow intermediate to form the acyl azolium intermediate and MeOH (100 eq) was added to quench acyl azolium intermediates to form the ester products (Fig. 5c ). In the redox process, the D-labeled site remained intact. The intensity of ester products 10 and 11 were detected by LC-HRMS, the intensity ratio of them was 99:1. In the same way, we carried out further studies to replace the large sterically hindered oxidant DQ A with bulky less oxidants 3,3’,5,5’-tetramethyl-[1,1’-bi(cyclohexylidene)]−2,2’,5,5’-tetraene-4,4’-dione (DQ B) and benzoquinone (BQ) to obtain the same esterification products ( 10 and 11 ). The intensity of products 10 and 11 were detected by LC-HRMS under same conditions, the ratios were 98:2 (DQ B as oxidant) and 97:3 (BQ as oxidant), with no obvious negative effects compared to using DQ A as oxidant. Steric hindrance is not an important factor for this chemoselective oxidation reaction. Disparity in redox properties of Breslow intermediates with different reaction sites is more likely to lead to selective oxidation, it suggested that the formation of acyl azolium intermediate 1a(D)-II was much faster than 1a(D)-II’ (Fig. 5c ). Additional density functional theory (DFT) calculations were performed to estimate the Gibbs free energy barriers of the oxidation of Breslow intermediates (Fig. 5d ). In the calculation, the less sterically hindered BQ was selected as the oxidant in order to exclude the effect of steric hindrance. It was found that the β-site Breslow intermediate (ΔG ≠ = 11.52 kcal/mol) was more easily oxidated than the α-site (ΔG ≠ = 20.79 kcal/mol). Furthermore, the non-covalent interactions (NCI) of the transition structures were analyzed. It was shown that only the π-π stacking interaction were found between BQ and Breslow intermediates in the transition state, and the transition state could be stabled by the weak interactions. Overall, the experimental observations and DFT calculations were consistent with the finding that the reducibility of the β-site Breslow intermediate was higher than that of α-site when steric bulk was not present. In the model reaction condition (such as Table 1 , entry 12), the yield of desired product 3a didn’t over 70%. Unfortunately, no obvious byproduct could be isolated by flash column chromatography. To well investigate the formation of byproduct in the model reaction, the additional experiments were carried out (Fig. 5e ). Comparing with the standard condition (Table 1 , entry 12), the D-labeled enedial 1a(D) was employed in the control experiment, and the reaction was determined by in situ LC-HRMS. Finally, some polymerized products were found in the reaction. It was normal that the D-labeled acyl azolium intermediate 1a(D)-II was formed in the reaction. However, the remaining aldehyde moiety of acyl azolium intermediate 1a(D)-II was activated by acyl azolium moiety, and reacted with Breslow intermediate to form dimer intermediate 1a(D)-III . Furthermore, the 1a(D)-III continuously reacted with another Breslow intermediate and oxidized to form trimer 1a(D)-IV . Comparing with non-labeled enedial 1a , all the D-labeled site remained intact, so that the reacted sites can be clearly identified by HRMS. The fragmentation of 1a-IV in liquid chromatography high resolution accurate mass spectrometer (LC-HRMS-MS) was investigated and reviewed. In order to further speculate the structure of the reaction byproducts, we found some possible intermediates, including 1a-II , etc. (see Supplementary Information ). The formation of dimer and trimer polymerized products indicated that high reactivity aldehyde moiety of acyl azolium intermediate 1a(D)-II can easily and indiscriminately react with other nucleophilic substrates or intermediates. Thus, desired product and byproduct were formed, which will lead to decrease the yield of desired products. This furo[2,3-b]pyrrole is a common structural motif widely found in natural products and drugs, we were interested in preliminary exploration of its bioactivity. The furo[2,3-b]pyrrole derivatives from our approach also exhibited biological activity in our research on novel pesticide development for crop protections. For example, many of our compounds showed good antibacterial activities against Xanthomonas axonopodis pv. citri (Xac) which can cause citrus canker and result in huge economic losses in the production of lemons, oranges and grapefruits. 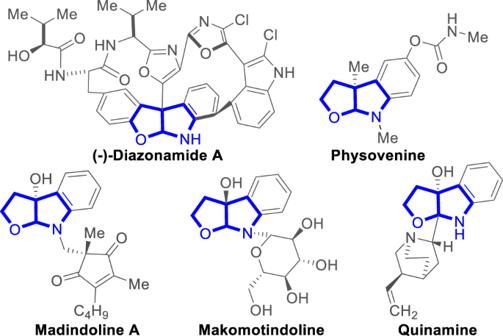Fig. 2: Functional molecules containing furo[2,3-b]pyrrole. Examples of functional chiral molecules. According to the analysis of Table 2 , it was found that substrates with ortho-F ( 3b ) and para-methoxy ( 3i ) substituents exhibited better activity when the enedials substrates were expanded. In addition, It was observed that when the methyl group was installed at the imine( 4i) exhibited good activity. Moreover, the derivatives 6, 7 and 8 from 3a , showed good activity exhibited good activity as well. Compared with the thiodiazole copper and bismerthiazo that have been widely used as commercially available antibacterial agrichemicals, some furo[2,3-b]pyrrole chiral molecules afforded from our method exhibited obviously superior antibacterial activities and can be regarded as promising candidates in the search for new pesticide lead compounds. Table 2 In vitro antibacterial activity of the target compounds against Xac a Full size table In summary, we have developed a chemo- and enantioselective strategy in transforming unsymmetric enedials to furo[2,3-b]pyrrole containing molecules. Our results suggested that the initial addition steps between the NHC catalyst and the aldehyde moieties of the enedial substate (to form the corresponding Breslow intermediates) do not provide sufficient differentiations on the two aldehyde moieties. Instead, the observed overall chemoselectivity was resulted from the Breslow intermediate oxidation event that offers a very significant chemoselectivity increase. Furthermore, multiple additional experiments were performed for the redox process, it was found that all the bulky or less bulky oxidants could be priority reducted by β-site Breslow intermediate, the observed overall chemoselectivity was resulted from the reducing properties of different sited Breslow intermediates. Multiple possible side reactions were elucidated by analyzing the reaction mixtures via LC-HRMS. The chiral furo[2,3-b]pyrroles derivatives from our reactions can be easily transformed into various functiona molecules. Further studies on the bioactivities of these chiral furo[2,3-b]pyrrole compounds for agricultural applications had been evaluated, the preliminary results suggested that these molecules show encouraging in vitro activities against Xac . Our method and its mechanistic implications shall also stimulate further reflect on driving force of chemoselective for the molecules bearing multiple structural units with similar reactivities. General procedure for the catalytic reactions To a dry 4.0 mL vial equipped with a magnetic stir bar, was added 1a (0.13 mmol), 2a (0.10 mmol), pre-NHC A (0.02 mmol), DQ A (0.13 mmol) and base (0.02 mmol). After purges with N 2 in glove-box, anhydrous MeCN (2.0 mL), and 4 Å MS (150.0 mg) was added and sealed. The reaction mixture was stirred at 45 °C for 12 h. Then the mixture was directly concentrated under reduced pressure to afford a crude product. 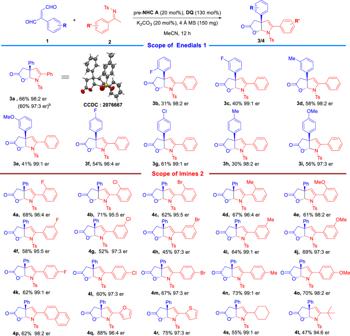Fig. 3: Substrates scope of the reactiona. aReaction conditions as stated in Table1, entry 12. Yields were isolated yields after purification by column chromatography. Er values were determined via HPLC on chiral stationary phase.bThe reaction was carried out at 1.0 mmol scale based on2a. 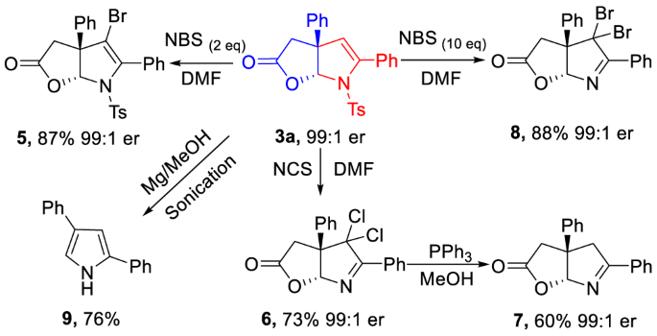Fig. 4: Synthetic transformations of 3a. Derivatization studies on3a. 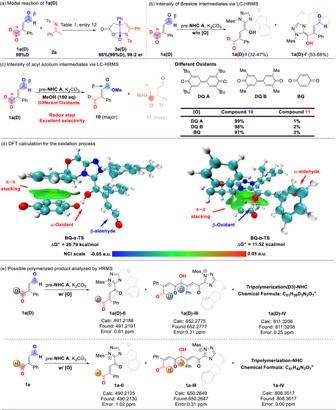Fig. 5: Additional supporting mechanistic experiments. aModel reaction of1a(D).bIntensity of Breslow intermediates via LC-HRMS.cIntensity of acyl azolium intermediates via LC-HRMS.dDFT calculation for the oxidation process.ePossible polymerized product analyzed by HRMS. The crude product was purified via column chromatography on silica gel (petroleum ether/ethyl acetate = 5/1) to afford the desired product 3a . Reporting summary Further information on research design is available in the Nature Portfolio Reporting Summary linked to this article.